Twisting phonons in complex crystals with quasi-one-dimensional substructures A variety of crystals contain quasi-one-dimensional substructures, which yield distinctive electronic, spintronic, optical and thermoelectric properties. There is a lack of understanding of the lattice dynamics that influences the properties of such complex crystals. Here we employ inelastic neutron scatting measurements and density functional theory calculations to show that numerous low-energy optical vibrational modes exist in higher manganese silicides, an example of such crystals. These optical modes, including unusually low-frequency twisting motions of the Si ladders inside the Mn chimneys, provide a large phase space for scattering acoustic phonons. A hybrid phonon and diffuson model is proposed to explain the low and anisotropic thermal conductivity of higher manganese silicides and to evaluate nanostructuring as an approach to further suppress the thermal conductivity and enhance the thermoelectric energy conversion efficiency. This discovery offers new insights into the structure-property relationships of a broad class of materials with quasi-one-dimensional substructures for various applications. Materials with a complex crystal structure continue to be the subject of a wide range of scientific studies and technological applications [1] , [2] . One particularly intriguing class of complex materials is those with quasi-one-dimensional (1D) substructures. Several notable examples of such materials are superconducting YBa 2 Cu 3 O 7−x (ref. 3 ), MoSe (ref. 4 ) and Li 0.9 Mo 6 O 17 (ref. 5 ) exhibiting Tomonaga-Luttinger liquid electronic properties, spin ladder or chain compounds with large directional magnon thermal conductivity [6] , and intermetallic Nowotny chimney ladder (NCL) phases [7] with potential technological applications in optoelectronic [8] and thermoelectric [9] , [10] devices. A prominent example of NCL phases is higher manganese silicides (HMS), Mn n Si 2 n − m , which consists of a tetragonal Mn chimney sublattice based on the β-Sn structure and a Si ladder sublattice with the atomic arrangement of coupled helices [11] . Each commensurate Mn n Si 2 n − m structure contains an integer number ( n ) of Mn sublattices and another integer number ( m ) of Si sublattices in one crystallographic unit cell. The crystal structures of four distinct phases have been reported, including the commensurate Mn 4 Si 7 phase shown in Fig. 1a and the Mn 11 Si 19 , Mn 15 Si 26 and Mn 27 Si 47 phases shown in Supplementary Fig. 1b . Each HMS phase exhibits nearly identical a lattice parameter and atomic ratio, but varying c lattice parameters, which can range from about 17 Å for Mn 4 Si 7 to as long as 118 Å for Mn 27 Si 47 . These phases are characterized by both local disorder and long range ordering, and sit at the transition from an ordered crystal to a disordered system. Such complex HMS structures exhibit low thermal conductivity ( κ ) and reasonably high thermoelectric figure of merit ZT = S 2 σT / κ , where S , σ and T are the Seebeck coefficient, the electrical conductivity and absolute temperature, respectively [11] . In contrast to most state-of-the-art thermoelectric materials such as lead telluride (PbTe), bismuth telluride (Bi 2 Te 3 ) and silicon germanium (SiGe), which contain rare, relatively costly, or toxic elements, HMS is made of two nontoxic elements that are abundant in the earth’s crust. The combination of such features has continued to drive the interest to better understand and further enhance the thermoelectric properties of HMS [11] , [12] , [13] , [14] , [15] , [16] , [17] . 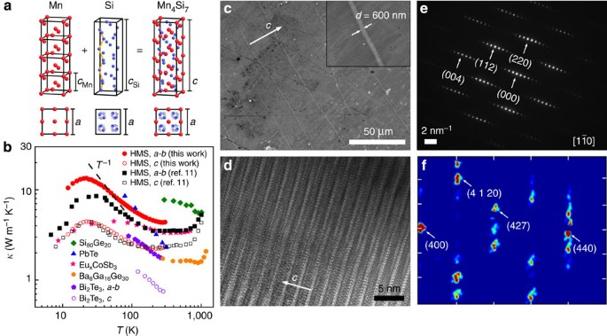Figure 1: Structure and thermal conductivity of higher manganese silicides. (a) Schematic illustrations of the crystal structure of Mn4Si7. The condition for a commensurate structure (MnnSi2n−m) satisfies the relationshipncMn=mcSi=cwherenandmare integers andc,cMnandcSiare the lattice constants along thecaxis for the HMS primitive cell, Mn sublattice and Si sublattice, respectively. (b) Temperature-dependent thermal conductivities of the HMS crystal measured in this work along thecandaaxes. Shown for comparison are the reported thermal conductivity data of HMS (ref.11), Bi2Te3(ref.18), PbTe (ref.19) and Ba8Ga16Ge30(ref.20) crystals, and Si80Ge20(ref.21) and EuxCoSb3(ref.22) alloys. (c) Scanning electron microscopy (SEM) image of the HMS crystal synthesized in this work. The inset is the magnified SEM image showing the presence of MnSi layers with a thickness of about 600 nm in the HMS crystal. (d) High-resolution transmission electron microscopy (HRTEM) lattice fringe image of the HMS region of the crystal. (e) Selected area electron diffraction (SAED) of the HMS crystal along thezone axis indexed with respect to the Mn sublattice. (f) Neutron diffraction pattern of the HMS crystal indexed with respect to the Mn27Si47phase. In both (e) and (f), the Si sublattice of a longcSiproduces characteristic satellite reflections along the [001] direction of the HMS crystal. Figure 1: Structure and thermal conductivity of higher manganese silicides. ( a ) Schematic illustrations of the crystal structure of Mn 4 Si 7 . The condition for a commensurate structure (Mn n Si 2 n − m ) satisfies the relationship nc Mn = mc Si = c where n and m are integers and c , c Mn and c Si are the lattice constants along the c axis for the HMS primitive cell, Mn sublattice and Si sublattice, respectively. ( b ) Temperature-dependent thermal conductivities of the HMS crystal measured in this work along the c and a axes. Shown for comparison are the reported thermal conductivity data of HMS (ref. 11 ), Bi 2 Te 3 (ref. 18 ), PbTe (ref. 19 ) and Ba 8 Ga 16 Ge 30 (ref. 20 ) crystals, and Si 80 Ge 20 (ref. 21 ) and Eu x CoSb 3 (ref. 22 ) alloys. ( c ) Scanning electron microscopy (SEM) image of the HMS crystal synthesized in this work. The inset is the magnified SEM image showing the presence of MnSi layers with a thickness of about 600 nm in the HMS crystal. ( d ) High-resolution transmission electron microscopy (HRTEM) lattice fringe image of the HMS region of the crystal. ( e ) Selected area electron diffraction (SAED) of the HMS crystal along the zone axis indexed with respect to the Mn sublattice. ( f ) Neutron diffraction pattern of the HMS crystal indexed with respect to the Mn 27 Si 47 phase. In both ( e ) and ( f ), the Si sublattice of a long c Si produces characteristic satellite reflections along the [001] direction of the HMS crystal. Full size image There is a lack of understanding of the lattice dynamics that influences the functional properties of these complex crystals with quasi-1D substructures. For example, one of the outstanding questions on HMS concerns the relationship between the complex NCL structure and the low and anisotropic thermal conductivity. As shown in Fig. 1b in comparison with other thermoelectric materials [11] , [18] , [19] , [20] , [21] , [22] , the thermal conductivity of HMS along the Si ladder direction ( c axis) can be a factor of two lower than that perpendicular to the ladder ( a axis). This κ anisotropy is similar in magnitude to layered Bi 2 Te 3 , where the heavy atoms are responsible for the inherently low κ and the large bonding anisotropy is responsible for the κ anisotropy [23] . As the bonding energy in HMS is not nearly as anisotropic as that in Bi 2 Te 3 , the reason for the κ anisotropy in HMS remains unclear. In addition, while nanostructuring has been successful in suppressing the lattice thermal conductivity ( κ L ) of some thermoelectric materials [24] , [25] , [26] , the origin of the already low κ in HMS bulk crystals needs to be better understood to evaluate the feasibility of further suppressing the thermal conductivity via nanostructuring. It has been suggested that low κ L can be achieved in crystals with a large and complex unit cell because a large fraction of phonon modes are optical modes with small group velocities and thus make little contributions to κ L (refs 27 , 28 ). However, the actual phonon dispersion, which is indispensable for understanding thermal transport, has remained unknown for HMS and other complex crystals with 1D substructures. Here we report inelastic neutron scattering (INS) measurements and density functional theory (DFT) calculations of the phonon dispersions in HMS crystals. The theoretical and experimental results reveal the presence of numerous low-lying optical vibration branches, especially a very low-lying optical phonon polarization associated with the twisting motions of the Si helices relative to the Mn chimney. In addition, the DFT calculations reveal higher group velocities for low-energy modes along the c axis than along the a axis, which is opposite to the thermal conductivity anisotropy, and a reversal of the group velocity anisotropy at an intermediate energy range. The results are used to establish a combined phonon and diffuson model to explain the thermal conductivity anisotropy in HMS crystals and to predict a glass-like thermal conductivity in nanostructured HMS. These findings shed light on the fascinating phonon dynamics in a broad class of complex materials with 1D substructures and a variety of functionalities. Structure characterization An HMS crystal rod with ∼ 6 mm diameter and 10 mm length was grown using the Bridgman method. As discussed in the Supplementary Methods , the X-ray diffraction (XRD) pattern of the HMS sample is matched best with that of the Mn 27 Si 47 phase, although the coexistence of other HMS phases is possible [29] . As shown in Fig. 1c , scanning electron microscopy (SEM) measurements reveal the presence of metallic MnSi lamellae, ∼ 600 nm wide and spaced ∼ 20 μm apart, which precipitate perpendicular to the c axis [10] . The presence of the MnSi phase has previously been reported in crystalline HMS samples [10] , and is caused by the peritectic decomposition of HMS. A high-resolution transmission electron microscopy (HRTEM) image ( Fig. 1d ) obtained from one HMS region shows modulated lattice fringes that are characteristics of the NCL superlattice [30] , [31] . The corresponding selected area electron diffraction (SAED) pattern ( Fig. 1e ) reveals parallel arrays of closely packed satellite peaks aligned along [001]. Produced by the long c Si , the satellite peaks are also discernible in the elastic neutron diffraction pattern shown in Fig. 1f . Inelastic neutron scattering measurements of phonons INS measurements of the four-dimensional scattering function, S ( Q ,E ), were performed on an HMS crystal sample at 300 K using both a time-of-flight wide angular-range chopper spectrometer (ARCS) [32] and a triple-axis spectrometer. 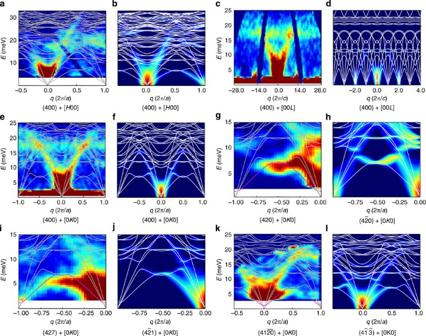Figure 2: Measured INS (ARCS) signal in comparison with simulated dynamical structure factor for the HMS crystal at 300 K. S(Q,E) data obtained by ARCS (a,c,e,g,i,k) for the HMS crystal and simulated dynamical structure factor (b,d,f,h,j,l) for Mn4Si7: (a,b) along [H00] in the (400) Brillouin zone, showing the LA and LO modes; (c,d) along [00L] in the (400) zone, showing mainly the TA and TO modes; (e,f) along [0K0] in the (400) zone, showing mainly thea-bpolarized TA and TO modes; (g,h) along [0K0] in the (420) zone, showing mainly thea-bpolarized TA and low lying optical modes; (i,j) along [0K0] in the (427) zone of Mn27Si47, showing the twisting and TA modes; (k,l) along [0K0] in thezone of Mn27Si47, showing mainly the twisting and TA modes. The white solid lines in all figures are the calculated harmonic dispersions of Mn4Si7. Becausem=1 and 7 for the Mn4Si7and Mn27Si47phases, respectively, the appropriate comparisons with the (427) andzones for Mn27Si47are the (421) andzones for Mn4Si7. In addition, the simulations of the (420), (421) andexhibit a mirror reflection with respect to the experimental data along [0K0]. As such, (h,j,l) show the simulations of the,andzones of Mn4Si7, as discussed inSupplementary Discussion. The calculated twisting polarization is labelled as the purple line ing,i,k. Different versions ofg,iwith energy up to 25 meV are shown asSupplementary Fig. 7. Figure 2 shows the experimental INS ARCS signal obtained from the HMS crystal with either 40 meV ( Fig. 2a,c,e ) or 30 meV ( Fig. 2g,i,k ) incident neutron energy along the phonon wave vector q =[ H 00], [0 K 0], and [00 L ] from different Brillouin zones, which are indexed by the reciprocal lattice vector G HKL =(400), (420), (427), and with respect to the Mn 27 Si 47 phase. Figure 2: Measured INS (ARCS) signal in comparison with simulated dynamical structure factor for the HMS crystal at 300 K. S ( Q , E ) data obtained by ARCS ( a , c , e , g , i , k ) for the HMS crystal and simulated dynamical structure factor ( b , d , f , h , j , l ) for Mn 4 Si 7 : ( a , b ) along [ H 00] in the (400) Brillouin zone, showing the LA and LO modes; ( c , d ) along [00 L ] in the (400) zone, showing mainly the TA and TO modes; ( e , f ) along [0 K 0] in the (400) zone, showing mainly the a - b polarized TA and TO modes; ( g , h ) along [0 K 0] in the (420) zone, showing mainly the a - b polarized TA and low lying optical modes; ( i , j ) along [0 K 0] in the (427) zone of Mn 27 Si 47 , showing the twisting and TA modes; ( k , l ) along [0 K 0] in the zone of Mn 27 Si 47 , showing mainly the twisting and TA modes. The white solid lines in all figures are the calculated harmonic dispersions of Mn 4 Si 7 . Because m =1 and 7 for the Mn 4 Si 7 and Mn 27 Si 47 phases, respectively, the appropriate comparisons with the (427) and zones for Mn 27 Si 47 are the (421) and zones for Mn 4 Si 7 . In addition, the simulations of the (420), (421) and exhibit a mirror reflection with respect to the experimental data along [0 K 0]. As such, ( h , j , l ) show the simulations of the , and zones of Mn 4 Si 7 , as discussed in Supplementary Discussion . The calculated twisting polarization is labelled as the purple line in g , i , k . Different versions of g , i with energy up to 25 meV are shown as Supplementary Fig. 7 . Full size image For a net momentum transfer from the incident neutron of Q = G HKL + q , the measured neutron scattering intensity increases with , where is the polarization vector of the i th atom in the unit cell for a particular phonon mode α ( Supplementary Methods ). Consequently, the phonon modes revealed in the ARCS data for the G HKL =(400) zone are predominantly the longitudinal modes with q along [ H 00] ( Fig. 2a ) and transverse modes polarized in the a - b plane with q along [00 L ] ( Fig. 2c ) and [0 K 0] ( Fig. 2e ). For all three crystal directions in the (400) zone, the INS data show both the presence of approximately linear acoustic branches and flat optical branches. The flat optical branches appear in the energy range between 10 and 25 meV, which is rather low compared with the optical phonon energy of ∼ 40 meV in Si (ref. 33 ). Along [ H 00] ( Fig. 2a ), the longitudinal acoustic (LA) branch intercepts longitudinal optical (LO) branches about halfway between the zone centre and zone boundary at ∼ 15 meV. In comparison, Fig. 2e shows that the a - b polarized transverse acoustic (TA) branch along [0 K 0], extends to ∼ 15 meV energy ( E ) and intercepts the a - b polarized transverse optical (TO) branches near the zone boundary. Remarkably, a broad linear band along [00 L ] ( Fig. 2c ) appears to extend to roughly 27π/ c or π/ c Mn , the zone boundary of the Mn sublattice instead of that of Mn n Si 2 n − m . As the component of Q in the a - b plane is increased towards the (420) zone ( Fig. 2g ), the measurement data along [0 K 0], which is expected to contain mainly a - b polarized transverse polarizations, reveals another branch that bends down to about 6 meV at the zone boundary. As the component of Q along the c axis is increased towards the (427) zone, modes with polarizations in both the a - b plane and c axis can contribute to the measurement data along [0 K 0] and [ H 00], namely Fig. 2i and Supplementary Fig. 5a , respectively. Both of these sets of data, especially the latter one, clearly reveal an additional low energy branch extending to the zone boundary at roughly 5 meV. As the component of Q along the c axis increases further towards the zone so that the measurement data are increasingly sensitive to c -polarized modes, the measurement data along [0 K 0] mainly contain two branches, one similar to the low energy branch shown in Fig. 2i and Supplementary Fig. 5a and the other with energy close to the a - b polarized TA branch of Fig. 2g . Density functional theory calculation of phonon dispersion To gain further insight into the INS measurement results and the phonon dispersion in HMS, we conducted DFT calculations of the phonon dispersion and electronic band structure of Mn 4 Si 7 ( Supplementary Discussion ). This simplest HMS phase shown in Fig. 1a has nearly seven times fewer atoms per unit cell than Mn 27 Si 47 , the majority phase determined for our HMS samples, which would require orders of magnitude more computation time than for the Mn 4 Si 7 phase. Nevertheless, the crystal structures of these two phases are still rather similar, except for minute differences in the Si ladder structure. 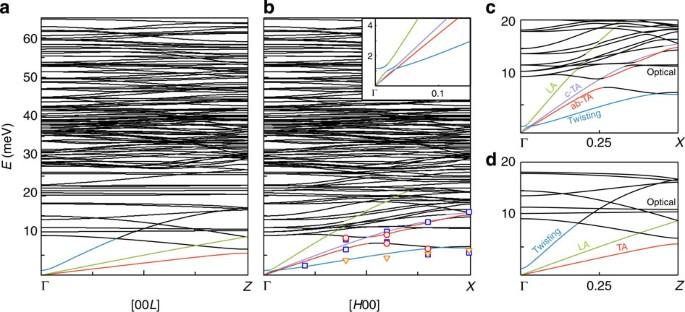Figure 3: Calculated phonon dispersion of Mn4Si7. (a,b) Calculated harmonic dispersions of Mn4Si7(solid black lines). The open symbols in (b) are the Gaussian fitting of the peak position of the INS line width measured with the triple-axis instrument at 300 K in the (200) zone (blue squares),zone (red circles) andzone (orange triangles) along [0K0]. (c,d) The calculated low-energy harmonic dispersions indexed by the polarization as LA, TA, twisting or other optical modes. The inset to (b) shows the modes close to the avoided crossing at∼1 meV along the Γ−X direction, with the color coding of the modes the same as that in (c). Figure 3 shows the calculated full-phonon dispersion along the two principal axes of Mn 4 Si 7 , [00 L ] and [ H 00], the latter of which is equivalent to [0 K 0]. The calculation results reveal numerous flat optical branches with energy as low as about 10 meV, in agreement with the experimental observations. The polarizations of the calculated phonon branches are determined according to an approach explained in Supplementary Discussion , and are shown in Fig. 3c,d . Figure 3: Calculated phonon dispersion of Mn 4 Si 7 . ( a , b ) Calculated harmonic dispersions of Mn 4 Si 7 (solid black lines). The open symbols in ( b ) are the Gaussian fitting of the peak position of the INS line width measured with the triple-axis instrument at 300 K in the (200) zone (blue squares), zone (red circles) and zone (orange triangles) along [0 K 0]. ( c , d ) The calculated low-energy harmonic dispersions indexed by the polarization as LA, TA, twisting or other optical modes. The inset to ( b ) shows the modes close to the avoided crossing at ∼ 1 meV along the Γ−X direction, with the color coding of the modes the same as that in ( c ). Full size image A significant finding from the calculation results is the discovery of the lowest-lying optical (LLO) polarization with energy comparable to the three acoustic polarizations. A video of the atomic motions of the LLO polarization is included in Supplementary Movie 1 , and shows a twisting motion of the Si atoms and a nearly stationary Mn sublattice with minor translations along the c axis. Such twisting modes are commonly associated with quasi-1D structures such as single-walled carbon nanotubes [34] , where they are purely acoustic modes. In the case of the Si helices interacting with adjacent helices and the Mn chimneys in the three-dimensional HMS structure, the twisting polarization is an optical branch with a nonzero energy of 0.8 meV at the zone centre, according to the calculation results shown in the inset of Fig. 3b . In addition, because of the anisotropic structure, the calculation results show that the two TA polarizations are degenerate along [00 L ] but slightly non-degenerate along [ H 00] and [0 K 0]. Because of the strong interaction between adjacent Si atoms within each helix, a high group velocity of 20.8 km s −1 at q =0.1(2π/ c ) along [00 L ] is calculated for the twisting mode ( Supplementary Table 1 ), which lies above the three acoustic polarizations along this direction. In comparison, the interaction between the adjacent Si helices is relatively weak. Consequently, the twisting polarization is the lowest energy polarization along [ H 00] and [0 K 0] except near the zone centre, where it undergoes two consecutive avoided crossings with the LA and c -polarized TA branches at a very low energy of about 1.4 meV, as illustrated in the inset of Fig. 3b and discussed in the Supplementary Discussion . In addition, the calculation suggests another avoided crossing of the a - b polarized TA branch and an optical branch near E =9 meV and q =0.25(2π/ a ) ( Fig. 3c ). Indicating a similar symmetry in the displacement patterns of two hybridized modes ( Supplementary Discussion ), avoided crossings of this kind have been observed between the rattler mode and acoustic modes in the clathrate β-Ba 8 Ga 16 Ge 30 (ref. 35 ), where the on-centre rattler was found to flatten the phonon branches instead of providing a strong phonon scattering mechanism. Theoretical analysis has further suggested that an avoided crossing with a low-lying optical polarization results in a wide, flat transverse acoustic branch in β-Ba 8 Ga 16 Sn 30 with off-centre rattlers, and that such flattening of the acoustic phonon dispersion results in a glass-like plateau in the thermal conductivity [36] , [37] . To compare the theoretical dispersion with the experimental INS results, we have further calculated the neutron scattering intensity from a given Brillouin zone, G HKL , using the theoretical harmonic dispersions ( Supplementary Discussion ). The results are presented in Fig. 2b,d,f,h,j,l . In general agreement with those measured by INS for the acoustic branches and low-energy optical modes, the simulated INS intensity results verify that the observed linear branch in Fig. 2a is the LA polarization along [ H 00]. Similarly, the broad linear band observed in Fig. 2c is due to TA and TO phonons along [00 L ]. In addition, the nearly linear branch observed from the (400) zone along the [0 K 0] direction in Fig. 2e contains only the a - b polarized TA modes, which exist on two separate branches before and after the avoided crossing with an optical branch at 9 meV ( Fig. 3c ). In comparison, for the (420) zone ( Fig. 2g ), the simulations suggest that the branch observed to bend down towards the zone boundary at 6 meV is an a-b polarized TO branch, which encounters an avoided crossing with the a - b polarized TA branch. The atomic motions corresponding to this optical mode are shown in Supplementary Movie 2 and discussed in Supplementary Discussion . For the (427) zone along [0 K 0] ( Fig. 2i ) and [ H 00] ( Supplementary Fig. 5a ) as well as the zone along [0 K 0] ( Fig. 2k ), the observed lowest-energy branch matches best the calculated twisting polarization, the simulated neutron intensity of which is one order of magnitude higher than that for the closest a - b polarized TA polarization. In addition, the a - b polarized TA branch has been observed experimentally in the (400) zone along [0 K 0] ( Fig. 2e ) at a higher energy than the low-energy branch observed in Fig. 2i,k and Supplementary Fig. 5a . It is important to note that because the c lattice parameter in the HMS unit cell is much larger than the a or b lattice parameter, a factor of 20 for Mn 27 Si 47 , a momentum transfer of still represents a fairly small momentum transfer in the [00 L ] direction. As a result, the c -polarized TA modes from this zone are expected to be masked by the much stronger intensity of the nearby a - b polarized TA modes. Hence, the lowest-energy branch observed in Fig. 2i,k along [0 K 0] and in Supplementary Fig. 5a along [ H 00] must be the twisting polarization. This conclusion is further supported by the additional triple-axis neutron scattering measurement results included in Fig. 3b , where the observed phonon peaks follow the calculated TA and twisting modes quite well. We note that the measured twisting mode frequencies are slightly lower than those calculated for the Mn 4 Si 7 phase. This difference can be attributed to the difference in the c lattice parameters of the HMS phases measured by INS and considered in the DFT calculation. The low frequencies of the twisting modes are associated with the large total mass of the long Si helices, and can decrease with increasing c lattice parameter or mass of the Si helices. We also note that INS measurements do not have sufficient resolution to reveal the fine features of the avoided crossing between the twisting polarization and the LA and c -polarized TA branch along the Γ−X direction. In addition, the zone centre energy of the twisting polarization is too low to be detected by INS or by far-infrared spectroscopy or Raman scattering measurements discussed in Supplementary Methods . Despite these limitations in existing experimental techniques, the presence of the lowest lying twisting polarization has been clearly identified by both the ARCS ( Fig. 2i,k , and Supplementary Fig. 5a ) and triple-axis measurement results ( Fig. 3b ). We have also measured the phonon density of states (DOS) with INS on HMS powder samples. As shown in Fig. 4a , the measured DOS is in good agreement with the calculated DOS determined from the calculated dispersion for Mn 4 Si 7 . However, in the high-energy range between 50 and 60 meV, the calculated DOS does not reveal the broad peak shown in the INS data in the HMS sample. One possible cause of this discrepancy is the variation in the high-energy optical modes associated with the slightly different Si ladder sublattices considered by the calculation and encountered in the experiment. Moreover, the strong anharmonicity can make the high-energy phonon spectrum deviate from the harmonic lattice dynamical calculation. The contributions to the specific heat from the LA modes, the two TA modes, the LLO or twisting modes, other optical modes, and electrons have been calculated and are shown individually in Fig. 4b . Because of the low energy of the numerous optical polarizations, their contribution to the specific heat is found to be dominant above 20 K. In comparison, for T <8 K, the total specific heat is dominated by the electronic specific heat calculated semi-classically based on the electronic band structure as implemented in BoltzTraP (ref. 38 ; see Supplementary Discussion for details). The calculated total specific heat compares well with the measured values. 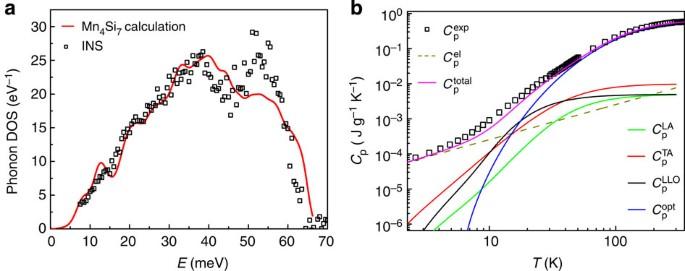Figure 4: Phonon DOS and specific heat. (a) Neutron weighted phonon DOS of HMS polycrystalline sample at 300 K compared with the calculated phonon DOS of Mn4Si7, which was corrected for neutron weighting. (b) Measured specific heatof an HMS crystal compared with the calculated specific heatof Mn4Si7. The calculated specific heat consists of the contributions from electron, LA modes, TA modes, twisting or LLO modesand other optical modes. Figure 4: Phonon DOS and specific heat. ( a ) Neutron weighted phonon DOS of HMS polycrystalline sample at 300 K compared with the calculated phonon DOS of Mn 4 Si 7 , which was corrected for neutron weighting. ( b ) Measured specific heat of an HMS crystal compared with the calculated specific heat of Mn 4 Si 7 . The calculated specific heat consists of the contributions from electron , LA modes , TA modes , twisting or LLO modes and other optical modes . Full size image Thermal conductivity model We now attempt to understand the anisotropic thermal conductivity of HMS based on the obtained phonon dispersion. The average group velocity components along the a and c axes are calculated from the phonon dispersion as a function of energy according to the method discussed in Supplementary Discussion . As shown in Fig. 5a , the obtained value is higher along the c axis than along the a axis for energy below ∼ 7 meV. Similarly, Supplementary Fig. 8 shows that the group velocities are higher along the c axis than along the a axis for the LA, TA and twisting polarizations at energies below about 7 meV, and that the group velocity anisotropy of the twisting polarization is most pronounced. However, the group velocity anisotropy is reversed at higher energies between ∼ 7 and ∼ 40 meV, because a larger c lattice parameter results in lower average group velocity components along the c axis than along the a axis for some optical modes. 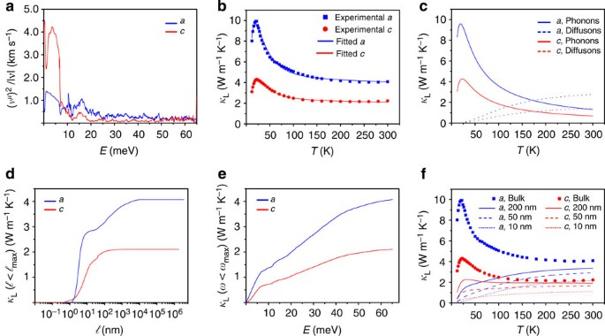Figure 5: Group velocity and lattice thermal conductivity calculations. (a) Calculated average group velocity components along theaandcaxes as a function of energy according to the method described inSupplementary Discussion. (b) The lattice thermal conductivity along theaandcaxes, as given by equation (1) with the fitted parameters stated in the text and compared with the lattice thermal conductivity of our sample. (c) The contributions to the lattice thermal conductivity from phonons and diffusons. (d) Accumulated lattice thermal conductivity at temperature 300 K from vibration modes with mean free path less thanℓ. (e) Accumulated contributions to lattice thermal conductivity at 300 K from vibrational modes with energy less thanE. (f) The lattice thermal conductivity as a function of temperature for various boundary scattering mean free paths. Figure 5: Group velocity and lattice thermal conductivity calculations. ( a ) Calculated average group velocity components along the a and c axes as a function of energy according to the method described in Supplementary Discussion . ( b ) The lattice thermal conductivity along the a and c axes, as given by equation (1) with the fitted parameters stated in the text and compared with the lattice thermal conductivity of our sample. ( c ) The contributions to the lattice thermal conductivity from phonons and diffusons. ( d ) Accumulated lattice thermal conductivity at temperature 300 K from vibration modes with mean free path less than ℓ . ( e ) Accumulated contributions to lattice thermal conductivity at 300 K from vibrational modes with energy less than E . ( f ) The lattice thermal conductivity as a function of temperature for various boundary scattering mean free paths. Full size image We next examine whether scattering is also anisotropic in HMS. The characteristic high-temperature plateau seen in the thermal conductivity curves [11] points to non-plane-wave-like behavior of some vibrational modes in these samples. As suggested by Zaitsev and Fedorov [39] , optical phonons in HMS and other complex crystals behave as those in an amorphous material. More specifically, scattering in the low-κ complex materials is expected to be intense so that the wave vector is no longer a well-defined parameter for vibrations with frequencies above a certain threshold known as the Ioffe-Regel crossover [40] , [41] . Only extended modes below the crossover behave as propagating phonons. In comparison, non-extended modes above the crossover can be neither propagating nor localized, and are referred to as diffusons according to the Allen-Feldman theoretical framework [40] , which suggests the occurrence of diffuson behaviour not only in glasses but also in both strongly disordered, crystalline solid solutions and weakly disordered crystals with very complicated unit cells. As HMS is a weakly disordered crystal with complex unit cells, we treat the non-extended vibrational modes as diffusons. This simple model has not taken into account strongly localized modes, which transport heat only via hopping caused by anharmonic coupling with extended modes [40] , [42] . Hence, the lattice thermal conductivity of HMS is expressed as sums of separate contributions from the phonon gas and diffusons, where α sums over all extended modes, q sums over all lattice vectors in the Brillouin zone, n is the Bose–Einstein distribution, τ α is the relaxation time for phonon mode ( q , α ), is the group velocity along direction μ , g d ( ω ) is the diffuson density of states and D μ ( ω ) is their diffusivity along direction μ . The INS measurements reveal well-defined phonon branches at energy up to about 20 meV, above which only flat broad intensity bands can be found. Therefore, we choose the cutoff between diffusons and propagating phonons as ω c =20 meV. Our model for the phonon relaxation time includes anharmonic and boundary contributions to scattering [43] , expressed in the following simple analytical form: where L is the boundary scattering mean free path in the bulk crystal sample, g p ( ω ) is the phonon density of states, and the min function is used to ensure that the anharmonic relaxation time is not lower than half of the oscillation, π / ω , consistent with the Ioffe–Regel limit [44] , [45] . For diffusons we assume a diffusivity D ( ω )= D 0 ω c / ω , which is consistent with the frequency dependence of the Ioffe–Regel limit. In this model, B , D 0 and L are taken as adjustable parameters for each direction and fitted to the lattice thermal conductivity determined from our experimental data. Further details about the model and the fit are provided as part of the Supplementary Discussion . As compared with the grey medium model with a constant mean free path, a non-grey model based on the actual dispersion and density of states is expected to improve the accuracy and agreement with the experimental results, as discussed in a recent work [46] . We obtain the values B =0.610 and 4.85 rad ps −2 , D 0 =3.50 and 1.79 nm 2 ps −1 , and L =18041 and 923 nm, respectively, along the a axis and c axis. As shown in Fig. 5b , the fit manages to satisfactorily reproduce our lattice thermal conductivity data along both axes. We note that our thermal conductivity values are nearly the same as the literature values [11] along the c axis, and somewhat higher than the literature values along the a axis. If the literature thermal conductivity values instead of our own results are used for the model fitting, the phonon relaxation time and diffusion coefficient would remain approximately the same for the c axis and reduce by about a factor of 0.7−0.8 for the a axis. The modelling results point to very anisotropic behavior of the propagating phonon modes and also some anisotropy in the diffusons. The values of D along both axes differ by a factor less than 2, whereas B and L change by about one order of magnitude between both directions. The much smaller B and much larger L values for the a axis are needed to overcome the smaller group velocity component of the low-frequency phonon modes along the a axis than along the c axis. Analysis of the propagating phonon and diffuson contributions to the lattice thermal conductivity ( Fig. 5c ) confirms that both contributions are anisotropic, with propagating phonon modes being chiefly responsible for the anisotropy at low temperatures and diffusons taking over around 150 K. Anisotropic phonon-boundary scattering can originate from the stacking of different phases in HMS. The co-existence of different HMS phases has been found in our XRD, HRTEM and SAED results as well as in previous works [29] , [31] . While the SEM image of Fig. 1c reveals some MnSi layers approximately perpendicular to the c axis and separated by about 20 μm distance, such surface measurements are not capable of detecting the MnSi layers buried under the surface as well as different HMS phases stacked perpendicular to the c axis caused by the modulation of the Si ladder [11] , [29] , [31] . The interfaces between different HMS and MnSi phases scatter phonons in a manner similar to phonon-boundary scattering in a thin film or a thin film superlattice structure, which has little effect on phonons travelling nearly parallel to the interface and making significant contribution to the in-plane heat current [47] , [48] , [49] , [50] . Consequently, boundary scattering alone is insufficient to yield a finite in-plane conductivity of a thin film. This effect allows for the in-plane component of the phonon mean free paths to be up to several orders of magnitude larger than the thickness of the film or the layers of the superlattice [47] , [48] , [49] , [50] , which limits the cross-plane component of the phonon-mean free path. Therefore, the much longer L found along the a axis can be understood as a consequence of the stacking of different MnSi and HMS phases perpendicular to the c axis. In addition, previous first principle calculations of Si and PbTe have found that the phonon life time at the same frequency and polarization can vary with the phonon wave vector by as much as one order of magnitude [51] , [52] . Compared with the relatively isotropic Si and PbTe structures, the atomic modulation along the long Si helices in HMS [31] results in a very narrow Brillouin zone along the c axis, which can significantly increase the umklapp scattering rate for phonons travelling along the c axis compared with that along the a axis. In addition, the anisotropic inter-atomic bonding arrangement in HMS may also give rise to some anisotropy in the diffusion coefficient for diffusons. Figure 5d clearly shows that most heat is carried by vibrational modes with mean free paths of 1–20 nm in HMS crystals at 300 K. Figure 5e presents the accumulated contributions to lattice thermal conductivity versus energy. It is found that even diffusons with rather high energies over 40 meV make considerable contribution to the room-temperature thermal conductivity, resulting in the observed high-temperature thermal conductivity plateaus. On the basis of the fitted lattice thermal conductivity of HMS crystals, we have calculated the κ L of nanostructured HMS by adding a grain boundary scattering contribution to the phonon scattering with a mean free path ℓ b . Details can be found in Supplementary Discussion . As shown in Fig. 5f , when ℓ b is reduced to about 10 nm, a reduction in κ L by as much as 45% or more at 300 K can be achieved to obtain a glass-like thermal conductivity. Even a grain size around 50 nm is sufficient to reduce κ L by about 25% at room temperature. The effect becomes more important at lower temperatures. For example, a ∼ 200 nm grain size causes a drop in κ L between 50% along the a axis and 20% along the c axis at T =100 K. This result suggests that lattice thermal transport in the HMS bulk crystal is dominated by phonons with rather long mean free paths at low temperatures. The different magnitude of the size effects along the two directions considered is caused by the very anisotropic behaviours of the phonon scattering in the bulk crystal. These experiments and calculations clearly reveal that the complex NCL structure of HMS gives rise to numerous low-lying optical vibration modes, including a peculiar twisting polarization that undergoes avoided crossings with the acoustic branches near the Brillouin zone centre. In additional to their low group velocities, these low-lying optical modes provide a large phase space for scattering of acoustic phonons. These features result in inherently low thermal conductivity of HMS. In addition, the calculation reveals a reversal of the group velocity anisotropy at energies above and below about 7−10 meV. In particular, minor modulations of the helical Si ladder between adjacent Mn sublattices result in lower average group velocity of some low-lying optical modes along the c axis compared with the a axis at energies above 10 meV as well as much more intense phonon scattering and somewhat lower diffusion coefficient along c , while distortions in the Si helices may lead to the stacking of different phases along the c axis and limit the boundary scattering mean free path component along the c axis. These observations help explain the considerable anisotropy in the thermal conductivity of HMS. Because low-frequency phonons with relatively long mean free path still makes considerable contribution to the thermal conductivity in HMS crystals according to a combined low-frequency phonon and high-frequency diffuson model, our calculation suggests that glass-like thermal conductivity is achievable by introducing grain boundary scattering with a length scale of about 10 nm. As the charge carrier mean free path of HMS is estimated to be about 1–2 nm based on a two band semi-classical model [12] , it is expected that the electrical properties of HMS would not be affected significantly by reducing the grain size to 10 nm. Therefore, a ZT larger than 1 is possible by nanostructuring HMS, as a ZT of 0.6–0.7 has been achieved in doped samples with grain size of several micrometres [13] , [14] , [16] . More broadly, the twisting polarization discovered in HMS gives the first glimpse of the elusive and important lattice dynamics in a wide range of complex crystals with promising functionalities as a result of internal quasi-1D substructures. Material synthesis and characterization An HMS crystal was grown by melting the powder sample via the Bridgman method. The crystal structure of the HMS samples was characterized via XRD using a Phillips X’pert diffractometer with the Cu K α radiation on the powder sample, which was made by crushing an HMS crystal. The morphology and chemical compositions of finely polished HMS samples were analysed with a Quanta 650 environmental SEM with an energy-dispersive X-ray (EDX) spectrometer. TEM, HRTEM and SAED of the samples were performed in a FEI Titan aberration-corrected (S)TEM electron microscope. The low-temperature thermal conductivity was measured by a steady-state method. The temperature-dependent specific heat data were collected using a 14-Tesla Quantum Design Physical Properties Measurement System in the temperature interval 1.9 K≤T≤300 K. Neutron scattering Measurements were conducted with the Wide Angular-Range Chopper Spectrometer (ARCS) at the Spallation Neutron Source at Oak Ridge National Laboratory (ORNL). The incident neutron energy was 40 or 30 meV with the sample maintained at room temperature and the beam incident on an HMS crystal mounted with the ( HK 0) crystallographic plane horizontal. Additional measurements were performed with the triple-axis spectrometer HB1 at ORNL. The DOS of a powder sample synthesized by solid-state reaction was measured with ARCS. Details of the measurements are given in Supplementary Methods . Theoretical calculations First-principles electronic structure calculations of Mn 4 Si 7 were performed using density functional theory within the generalized gradient approximation. The Perdue-Burke-Erznerhof (PBE) form was used for the exchange-correlation functional. The projector-augmented [53] , [54] plane wave basis method as implemented in VASP 5.3 (refs 55 , 56 ) was used for all structural relaxations and supercell calculations for interatomic force constants. A 4 × 4 × 2 Monkhorst-Pack k-point grid and a plane wave energy cutoff of 550 eV was used for all structural relaxations. The convergence threshold for energy and forces was set to 10 −6 eV and 10 −3 eV/Å, respectively. Phonon dispersions were determined using a real-space supercell approach. Ab initio force constant calculations were done using Phonopy [57] on a 2 × 2 × 2 supercell with a 2 × 2 × 1 q -point mesh, 500 eV energy cutoff and a higher 10 −8 eV energy convergence threshold. How to cite this article: Chen, X. et al. Twisting phonons in complex crystals with quasi-one-dimensional substructures. Nat. Commun. 6:6723 doi: 10.1038/ncomms7723 (2015).